Separate neural representations for physical pain and social rejection Current theories suggest that physical pain and social rejection share common neural mechanisms, largely by virtue of overlapping functional magnetic resonance imaging (fMRI) activity. Here we challenge this notion by identifying distinct multivariate fMRI patterns unique to pain and rejection. Sixty participants experience painful heat and warmth and view photos of ex-partners and friends on separate trials. FMRI pattern classifiers discriminate pain and rejection from their respective control conditions in out-of-sample individuals with 92% and 80% accuracy. The rejection classifier performs at chance on pain, and vice versa. Pain- and rejection-related representations are uncorrelated within regions thought to encode pain affect (for example, dorsal anterior cingulate) and show distinct functional connectivity with other regions in a separate resting-state data set ( N =91). These findings demonstrate that separate representations underlie pain and rejection despite common fMRI activity at the gross anatomical level. Rather than co-opting pain circuitry, rejection involves distinct affective representations in humans. The neural and psychological mechanisms of social rejection are the subject of intense study [1] , [2] , [3] , [4] , [5] ; rejection is experienced as painful , and is an important risk factor for physical and mental illnesses [6] , [7] and other functional impairments [8] . How rejection experiences are represented in the brain has great theoretical significance for understanding social and emotion processes [9] and translational implications for assessing and treating medical conditions influenced by social factors [10] , [11] . The ‘shared representation’ theory of social pain, the most influential theory of adverse social experience, suggests that rejection and related experiences piggyback on brain systems evolved to represent physical pain [1] , [2] , [3] . Experiences of social rejection and physical pain indeed have many common psychological and biological attributes. For example, both are often described using very similar words [1] and involve similar biological regulatory systems, such as endogenous opioids and oxytocin [12] , [13] . Critically, recent functional magnetic resonance imaging (fMRI) findings suggest that physical pain and social rejection activate common brain regions. These findings have been interpreted as evidence that pain and rejection share common brain representations [2] , [4] , [5] . Although the ‘shared representation’ theory does not claim that the neural systems underlying pain and rejection are exactly the same, it claims that shared representations exist in the brain regions thought to represent affective and sensory information in a modality-independent way. These regions include those important for representing affective distress across many conditions (for example, the dorsal anterior cingulate [dACC] and anterior insula [aINS]) [2] , [14] , [15] , [16] and those that represent somatosensory information more specifically (for example, dorsal-posterior insula [dpINS] and S2) [4] , [5] . However, overlapping fMRI activity within these regions does not necessarily imply shared representations at all levels of analysis (for example, neuronal population codes) [17] , [18] , [19] . For example, dACC and aINS show similar fMRI activity during the experience of positive and negative emotions [20] and also during diverse sensory and cognitive processes that have little to do with pain or rejection [21] , [22] . Thus, fMRI-based summaries of these regions often focus on potential common functions, such as surprise [23] or salience [24] . However, the dACC contains multiple, functionally specific subpopulations of neurons [25] , including nociceptive-specific ones [26] and those that code for various motivationally relevant events, such as reward expectancy [27] or predicted cognitive demands [28] . Even if the fMRI activity evoked by pain, rejection and other states is overlapping, their underlying neural representations may be non-overlapping. Thus, the question of whether representations of pain and rejection within dACC, aINS, dpINS, and S2 are common or distinct is unresolved. In this paper, we take a fresh look at the question of shared neural representations for pain and rejection, using multivariate pattern analysis (MVPA) [29] combined with a rigorous inferential logic, the ‘separate modifiability’ criterion [30] , for assessing shared versus distinct representations at the fMRI multivariate pattern level. The ‘separate modifiability’ criterion requires two different measures (here, two fMRI multivariate patterns) to be separately modulated by two manipulations without cross-influences. For example, if two fMRI multivariate patterns can be identified such that one pattern responds to manipulations of pain but not rejection, and the other pattern responds to rejection but not pain, the patterns are separately modifiable [30] . This criterion is well suited for ruling out a single-process account of function, such as intensity or salience. The rationale for this is laid out in detail in the Discussion and ref. 30 , but briefly, if two brain measures are separately modified by the two manipulations, then no single process is sufficient to account for the results. Therefore, separate modifiability can provide strong evidence for the existence of distinct brain representations for pain and rejection. We examined the following three specific questions in this paper: (i) whether global and local multivariate fMRI patterns that are separately modifiable by pain and rejection can be identified ( aim 1 ), (ii) whether or not those multivariate patterns for pain and rejection are correlated within and across regions ( aim 2 ) and (iii) whether the multivariate patterns for pain and rejection engage distinct functional brain networks ( aim 3 ). Even if standard fMRI activation is insufficient to capture activity in distinct neural circuits, multivariate patterns of fMRI activity may be able to capture neuronal population codes specific to distinct sensory and affective experiences [17] , [31] , [32] . Thus, it may still be possible to identify multivariate patterns that respond only to manipulations of pain or rejection, and thus demonstrate separate modifiability of the two processes within and across brain regions. In Study 1, 60 participants were scanned with fMRI while they experienced physical pain and social rejection stimuli on separate trials ( Fig. 1a ). We recruited individuals who recently experienced an unwanted break-up with their romantic partners and felt intensely rejected. In the social rejection task, in order to elicit emotions of social rejection, participants viewed a headshot photograph of their ex-partner (‘Ex-partner’ condition) or a close friend (‘Friend’ condition). In the somatic pain task, we delivered painful heat (‘Heat-pain’ condition) or warm heat (‘Warmth’ condition) to the left volar forearm. Data from part of this sample ( N =40) were previously published [4] , [32] , but the analyses we performed here are qualitatively different from those in previous reports; here we focus on identifying an fMRI multivariate pattern for rejection and assessing its relationship with somatic pain representations (see Discussion for additional details). 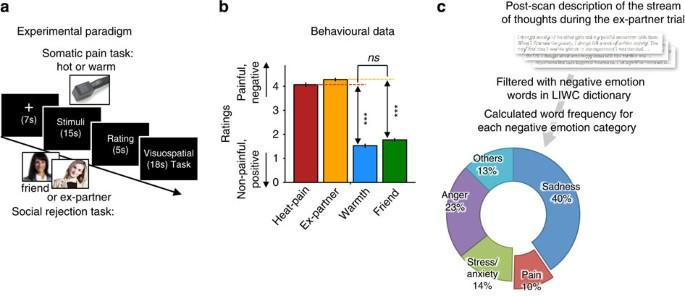Figure 1: Behavioural results. (a) Experimental paradigm. The social rejection and somatic pain tasks each consisted of two consecutively administered runs of eight trials (that is, 16 total trials). The order of the two tasks was counterbalanced across participants. (i) Social rejection task: each trial in the social rejection task lasted 45 s and began with a 7-s fixation cross. Subsequently, participants saw a headshot photograph of their ex-partner (‘Ex-partner’ condition) or a close friend (‘Friend’ condition) for 15 s. A cue-phrase beneath each photo directed participants to think about how they felt during their break-up experience with their ex-partner or a specific positive experience with their friend. Subsequently, participants rated how they felt using a five-point scale. To reduce carryover effects between trials, participants then performed an 18-s visuo-spatial control task in which they saw an arrow pointing left or right and were asked to indicate which direction the arrow was pointing. Ex-partner versus Friend trials were randomly presented with the constraint that no trial repeated consecutively more than twice. (ii) Somatic pain task: the structure of somatic pain trials was identical to rejection trials with the following exceptions. During the 15-s thermal stimulation period, participants viewed a fixation cross and focused on the sensations they experienced during a hot (painful) or warm (non-painful) stimulus that was delivered (1.5-s temperature ramp up/down, 12 s at peak temperature) to their left volar forearm at temperatures calibrated for each person (for details, see Methods). They then rated the pain they experienced using a five-point scale. (b) Behavioural data from trial-by-trial pain and emotion rating (n=60, eight trials for each condition). Error bars represent within-subject standard errors of the mean (s.e.m.). (c) Relative word frequency for negative emotion word categories among negative emotional words that participants used to describe the stream of thoughts while they were viewing the ex-partner’s photo in the scanner after the fMRI scanning. We used the Linguistic Inquiry and Word Count dictionary33(LIWC) to categorize emotional words. ***P<0.001, multi-level generalized linear model. Figure 1: Behavioural results. ( a ) Experimental paradigm. The social rejection and somatic pain tasks each consisted of two consecutively administered runs of eight trials (that is, 16 total trials). The order of the two tasks was counterbalanced across participants. (i) Social rejection task: each trial in the social rejection task lasted 45 s and began with a 7-s fixation cross. Subsequently, participants saw a headshot photograph of their ex-partner (‘Ex-partner’ condition) or a close friend (‘Friend’ condition) for 15 s. A cue-phrase beneath each photo directed participants to think about how they felt during their break-up experience with their ex-partner or a specific positive experience with their friend. Subsequently, participants rated how they felt using a five-point scale. To reduce carryover effects between trials, participants then performed an 18-s visuo-spatial control task in which they saw an arrow pointing left or right and were asked to indicate which direction the arrow was pointing. Ex-partner versus Friend trials were randomly presented with the constraint that no trial repeated consecutively more than twice. (ii) Somatic pain task: the structure of somatic pain trials was identical to rejection trials with the following exceptions. During the 15-s thermal stimulation period, participants viewed a fixation cross and focused on the sensations they experienced during a hot (painful) or warm (non-painful) stimulus that was delivered (1.5-s temperature ramp up/down, 12 s at peak temperature) to their left volar forearm at temperatures calibrated for each person (for details, see Methods). They then rated the pain they experienced using a five-point scale. ( b ) Behavioural data from trial-by-trial pain and emotion rating ( n =60, eight trials for each condition). Error bars represent within-subject standard errors of the mean (s.e.m.). ( c ) Relative word frequency for negative emotion word categories among negative emotional words that participants used to describe the stream of thoughts while they were viewing the ex-partner’s photo in the scanner after the fMRI scanning. We used the Linguistic Inquiry and Word Count dictionary [33] (LIWC) to categorize emotional words. *** P <0.001, multi-level generalized linear model. Full size image Through a series of analyses, we challenge the ‘shared representation’ theory by identifying whole-brain fMRI multivariate patterns separately modifiable by pain and rejection. In addition to separate modifiability at the whole-brain level, multivariate patterns coding for pain and rejection within the dACC, aINS, dpINS, and S2 are uncorrelated and separately modifiable. Resting-state connectivity analyses on a separate sample (Study 2, N =91) reveal that two multivariate patterns for pain and rejection encoded in the same set of dACC voxels have distinct functional connectivity patterns with the rest of the brain. These findings suggest that pain and rejection are distinct types of affect, with independent representations co-localized in similar gross anatomical regions. Behavioural results In Study 1, both the Heat-pain and Ex-partner conditions elicited substantial negative affect on numerical rating scales ( M Heat-pain =4.07±0.55 (s.d. ); M Ex-partner =4.28±0.39 on a five-point scale), compared with their respective control (Friend and Warmth) conditions, t Heat-pain versus Warmth (59)=29.07, P <0.001, t Ex-partner versus Friend (59)=28.37, P <0.001. Pain and rejection manipulations elicited equally strong increases in negative affect (for Heat-pain versus Ex-partner, , t (118)=0.26, P =0.80). Participants provided verbal descriptions of their experiences while viewing their ex-partner’s photo after the experiment. A word frequency analysis of these descriptions using the LIWC2007 software [33] revealed that, as expected, the photos elicited painful emotions: 9.7% of all negative emotion words provided by participants were pain-related words (for example, painful, hurt and so on), with 23% of participants using at least one pain-related word. The photos also evoked other negative emotions, including sadness (for example, sad, cry; 40.3% of negative emotion words used, and 85% of participants), anger (for example, angry, mad; 23.3% of negative emotion words, and 97% of participants) and stress (for example, upset, confused; 14.2% of negative emotion words, and 77% of participants). Thus, rejection-related stimuli did not only evoke ‘painful’ experiences, but they also elicited multiple intense, negative emotions. Separate modifiability of fMRI pattern-based classifiers To identify multivariate patterns of fMRI activity that are separately modifiable by pain and rejection ( aim 1 ), we trained linear support vector machines (SVMs) [34] to discriminate Heat-pain versus other conditions and Ex-partner versus other conditions with a leave-one-subject-out cross-validation [35] . We used whole-brain activation parametric maps that were masked by an a priori meta-analytic map associated with ‘pain’, ‘emotion’ and ‘social’ [22] (see Methods and Supplementary Fig. 1 ). In order to identify pain- and rejection-specific activation patterns if they exist, it is desirable to train the classifier on Heat-pain versus all other conditions (including Ex-partner) or Ex-partner versus others (including Heat-pain) rather than Heat-pain versus Warmth and Ex-partner versus Friend because the latter contrasts could capture signal from a single process, such as salience or general aversiveness. With the identified patterns for pain and rejection, we tested for separate modifiability by testing them on out-of-sample participants for Heat-Pain versus Ex-partner or Ex-Partner versus Heat-Pain, Heat-Pain versus Warmth and Ex-partner versus Friend contrasts. As shown in Fig. 2a and Supplementary Fig. 2 , the pain classifier discriminated Heat-pain versus Ex-partner with 100% accuracy in the test participants (95% confidence interval (CI): 100–100%, P <0.00001) and Heat-pain versus Warmth with 92% accuracy (CI: 84–99%, P <0.00001). However, it performed at chance for Ex-partner versus Friend (accuracy=59%, with 95% CI: 47–72%, P =0.193), demonstrating responsivity only to somatic pain. The rejection classifier discriminated Ex-partner versus Heat-pain with 88% accuracy (95% CI: 80–96%, P <0.00001) and Ex-partner versus Friend with 80% accuracy (95% CI: 69–90%, P <0.00001). However, it performed at chance for Heat-pain versus Warmth (accuracy=59%, with 95% CI: 47–72%, P =0.193), demonstrating responsivity only to rejection. These findings provide the first evidence for separate modifiability of whole-brain fMRI multivariate patterns for pain and rejection, suggesting the existence of functionally independent neural representations for pain and rejection. 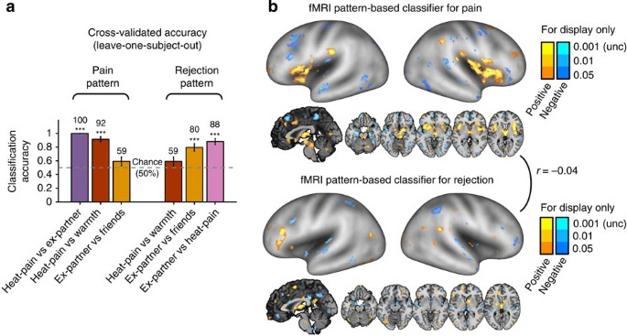Figure 2: Separate modifiability of fMRI pattern-based classifiers for pain and rejection. (a) Cross-validated (leave-one-subject-out) accuracy in two-choice classification tests (n=59). The results demonstrated separate modifiability (each can be changed independent of the other) of the fMRI pattern-based classifiers. The dashed line indicates the chance level (50%), and the error bars represent standard error of the mean across subjects. (b) The distributed fMRI pattern maps in which voxel activity reliably contributes to the discrimination of pain (top panel) and rejection (bottom panel) from other conditions. The maps show thresholded voxel weights based on bootstrapping (10,000 samples) of SVMs for display only; all weights were used in classification.rbetween two pattern maps denotes Pearson’s correlation of voxel weights. ***P<0.001, binomial test. Figure 2: Separate modifiability of fMRI pattern-based classifiers for pain and rejection. ( a ) Cross-validated (leave-one-subject-out) accuracy in two-choice classification tests ( n =59). The results demonstrated separate modifiability (each can be changed independent of the other) of the fMRI pattern-based classifiers. The dashed line indicates the chance level (50%), and the error bars represent standard error of the mean across subjects. ( b ) The distributed fMRI pattern maps in which voxel activity reliably contributes to the discrimination of pain (top panel) and rejection (bottom panel) from other conditions. The maps show thresholded voxel weights based on bootstrapping (10,000 samples) of SVMs for display only; all weights were used in classification. r between two pattern maps denotes Pearson’s correlation of voxel weights. *** P <0.001, binomial test. Full size image Figure 2b displays the classifier voxel weights that reliably contribute to the classification of pain and rejection, respectively, based on bootstrap tests with 10,000 iterations (thresholded at P <0.001 uncorrected for display only; all voxel weights were used in classification). Heat-pain versus Warmth was predicted by activation in many regions associated with nociceptive processing and endogenous pain control [36] , [37] , such as right (contralateral) dpINS, bilateral S2, medial thalamus and periaqueductal gray (PAG). Ex-partner versus Friend was predicted by increased activity in dorsomedial prefrontal cortex (dmPFC), right temporal parietal junction (TPJ) and precuneus, which are reliably associated with mentalizing about others [38] , [39] , and several other regions associated with negative emotion and its regulation [20] , [40] , [41] , including thalamus, supplementary motor area and inferior frontal gyrus. To statistically compare the two pattern maps for pain and rejection ( aims 2, 3 ), we conducted a bootstrap test with 10,000 iterations: for each iteration, we trained linear SVMs for pain and rejection and calculated (i) their spatial correlation across voxel weights and (ii) the difference weight values at each voxel. The two pattern classifiers were uncorrelated with each other, r =−0.04, P =0.28, and showed different weights in the following brain regions: Activation was more strongly predictive of pain in the supramarginal gyrus, middle insula, dpINS and ventral insula, PAG, amygdala and thalamus ( warm colours in Fig. 3a , q <0.05, false discovery rate [FDR] corrected; for the full list of the regions, see Supplementary Table 1 ). Activation was more strongly predictive of social rejection in dmPFC, right inferior frontal gyrus, ventromedial prefrontal cortex, perigenual anterior cingulate cortex, TPJ and precuneus ( cool colours in Fig. 3a ). The significant weight differences in these regions were mainly driven by significant positive weights for pain or rejection ( Fig. 3b ), but in some regions by significant negative weights; in particular, by negative weights for rejection in amygdala and thalamus. 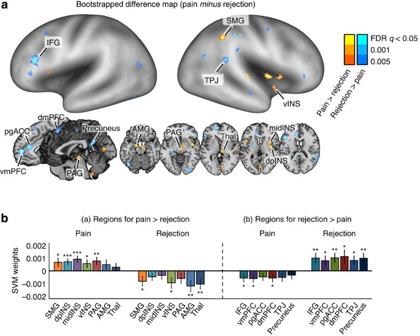Figure 3: The difference map between the fMRI pattern-based classifiers for pain and rejection. (a) The difference map in which values represent reliable differences between two discriminant weights (SVM weights for painminusSVM weights for rejection) based on bootstrapping of SVMs (10,000 samples). The difference map is thresholded atq<0.05, FDR corrected. AMG, amygdala; dpINS, dorsal posterior insula; IFG, inferior frontal gyrus; midINS, middle insula; PAG, periaqueductal gray; pgACC, pregenual anterior cingulate cortex; preSMA, pre-supplementary motor area; SMG, supramarginal gyrus; Thal, thalamus; TPJ, temporal parietal junction; vINS, ventral insula; vmPFC, ventromedial prefrontal cortex. (b) Mean SVM weights for contiguous regions within the difference map (10,000 samples). The error bars represent standard error of the mean based on bootstrapping. *P<0.05, **P<0.01, ***P<0.001, one-samplet-test. Figure 3: The difference map between the fMRI pattern-based classifiers for pain and rejection. ( a ) The difference map in which values represent reliable differences between two discriminant weights (SVM weights for pain minus SVM weights for rejection) based on bootstrapping of SVMs (10,000 samples). The difference map is thresholded at q <0.05, FDR corrected. AMG, amygdala; dpINS, dorsal posterior insula; IFG, inferior frontal gyrus; midINS, middle insula; PAG, periaqueductal gray; pgACC, pregenual anterior cingulate cortex; preSMA, pre-supplementary motor area; SMG, supramarginal gyrus; Thal, thalamus; TPJ, temporal parietal junction; vINS, ventral insula; vmPFC, ventromedial prefrontal cortex. ( b ) Mean SVM weights for contiguous regions within the difference map (10,000 samples). The error bars represent standard error of the mean based on bootstrapping. * P <0.05, ** P <0.01, *** P <0.001, one-sample t -test. Full size image Multi-voxel pattern similarity analysis Pain and rejection-related patterns included significantly different weights in some known targets of ascending nociceptive pathways [42] , including dpINS, thalamus and PAG, but not others (for example, dACC, aINS and S2). All of these regions were activated in standard general linear model (GLM) analyses by both Heat-pain versus Warmth and Ex-partner versus Friend contrasts ( Supplementary Fig. 3 ). Common GLM activations such as these results have been interpreted in terms of shared neural representations between pain and rejection in previous papers [2] , [3] , [4] . For this reason, and to identify shared local representations if they exist ( aim 2 ), we examined whether the individual patterns of fMRI activity within these nociceptive pain-processing regions were similar or different for each participant with multi-voxel pattern similarity analysis [17] , [43] . The pattern correlations within dACC, aINS, S2 and dpINS were calculated for each individual participant (i) between the SVM weights for pain and rejection across voxels, and (ii) between the first-level contrast activation maps for Heat-pain versus Warmth and Ex-partner versus Friend (see Supplementary Fig. 4 for the detailed analysis procedure). 95% CIs and P -values were calculated based on bootstrap tests with 10,000 iterations (for the correlations between SVM weights) or based on group statistics (for the correlation between contrast images). Pattern similarity analysis results supported the conclusion that pain- and rejection-related representations within pain-processing regions were distinct ( Fig. 4a ). No core pain-processing regions showed a significant correlation between (i) SVM classifier weights for pain and rejection ( Fig. 4b , left) or (ii) fMRI contrast images for pain and rejection ( Fig. 4b , right). Use of rank correlations yielded the same results. 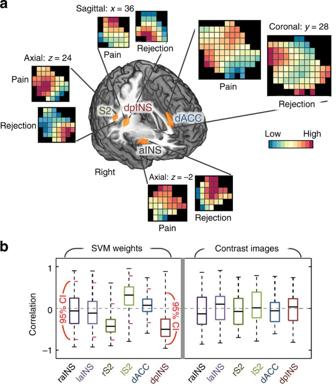Figure 4: Multi-voxel pattern similarity analysis for pain-processing regions. (a) SVM classifier weight patterns within regions-of-interest (ROIs) from group-level GLM results. The regions were activated in both contrasts, Heat-pain versus Warmth and Ex-partner versus Friend, and have been implicated in both pain and rejection. Here, a liberal threshold (P<0.05, uncorrected) was applied to use large enough regions for multi-voxel pattern similarity analyses (the averaged number of voxels across six ROIs=213). For GLM results corrected for multiple comparisons, seeSupplementary Fig. 3. The patterns presented here are the averaged SVM classifier weights from bootstrap tests (10,000 samples). aINS, anterior insula; dACC, dorsal anterior cingulate cortex; dpINS, dorsal posterior insula; S2, secondary somatosensory cortex. (b) Left: the bootstrap test results for SVM classifier weight correlations. Right: the group-level correlations between fMRI activations of contrast images for pain and rejection (n=59). The short red lines in the left panel indicate 95% confidence intervals obtained from bootstrap tests (10,000 samples). No regions showed significant correlations between SVM classifier weights, and no regions showed significant average correlations between patterns of contrast values across participants. Figure 4: Multi-voxel pattern similarity analysis for pain-processing regions. ( a ) SVM classifier weight patterns within regions-of-interest (ROIs) from group-level GLM results. The regions were activated in both contrasts, Heat-pain versus Warmth and Ex-partner versus Friend, and have been implicated in both pain and rejection. Here, a liberal threshold ( P <0.05, uncorrected) was applied to use large enough regions for multi-voxel pattern similarity analyses (the averaged number of voxels across six ROIs=213). For GLM results corrected for multiple comparisons, see Supplementary Fig. 3 . The patterns presented here are the averaged SVM classifier weights from bootstrap tests (10,000 samples). aINS, anterior insula; dACC, dorsal anterior cingulate cortex; dpINS, dorsal posterior insula; S2, secondary somatosensory cortex. ( b ) Left: the bootstrap test results for SVM classifier weight correlations. Right: the group-level correlations between fMRI activations of contrast images for pain and rejection ( n =59). The short red lines in the left panel indicate 95% confidence intervals obtained from bootstrap tests (10,000 samples). No regions showed significant correlations between SVM classifier weights, and no regions showed significant average correlations between patterns of contrast values across participants. Full size image Cross-classification test results with local classifiers Although pain- and rejection-related fMRI patterns were uncorrelated within core pain-processing regions, this does not imply that there are no shared representations anywhere in the brain. To identify regions with shared and non-shared local patterns between pain and rejection ( aims 1, 2 ), we conducted ‘cross-classification’ tests using a local pattern-based classification approach ( cf . ref. 44 ). The cross-classification tests consisted of three steps. (i) Local regions were defined using spherical searchlight regions around centre voxels [45] or using functional parcellations [46] . (ii) Multivariate pattern classifiers using a defined local region were trained separately for Heat-Pain versus Warmth and Ex-partner versus Friend with leave-one-subject-out cross-validation. In this analysis, training classifiers on one condition versus its control condition is more desirable than the one condition versus all other conditions approach because here we sought to identify ‘shared’ local representations across pain and rejection, not specific and unique representations of pain and rejection. (iii) With the identified local patterns for pain and rejection, we tested for separate modifiability by applying them to out-of-sample participants for the Heat-Pain versus Warmth and Ex-partner versus Friend contrasts. Steps ii and iii were repeated for each local region across the whole brain. If neural representations for pain and rejection are shared within a local region, the cross-validated accuracy for each classifier should be significant for both within- and cross-modality test contrasts. For example, a pattern trained on Heat-Pain versus Warmth would classify above chance for both Heat-Pain versus Warmth (within-modality) and Ex-partner versus Friend (cross-modality) in out-of-sample participants. To assess the robustness of the procedure across variations in the method, we conducted the cross-classification tests with four different local region definitions, including 6- and 10-mm radius spherical searchlights [45] , and 200- and 400-region functional parcellations [46] . As the results were comparable across all local region definitions ( Supplementary Fig. 5 ), here we focus on the results of 6-mm radius spherical searchlights ( Fig. 5 and Supplementary Fig. 6 ). 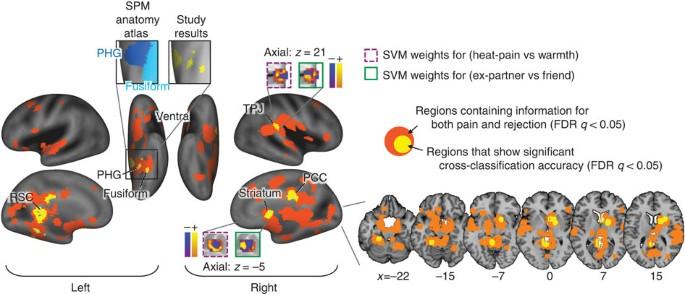Figure 5: Cross-classification test results with local pattern classifiers. We conducted whole-brain searches for candidate regions for shared neural processes between pain and rejection with 6-mm radius spherical searchlights around centre voxels. To determine the candidate regions, we conducted cross-classification tests (with leave-one-subject-out cross-validation) among the regions that accurately classify both pain (Heat-pain versus Warmth) and rejection (Ex-partner versus Friend). The cross-classification test consisted of the following steps: (i) A local classifier was trained and cross-validated separately for one condition, and (ii) the classifier was tested on the other condition in the same leave-one-subject-out cross-validation test sample. Here we thresholded all results at FDRq<0.05 (P<0.0038) and visualized the 6-mm sphere coverage. PCC, posterior cingulate cortex; PHG, parahippocampal gyrus; RSC, retrosplenial cortex; TPJ, temporal parietal junction. The anatomical atlas was from the SPM anatomy toolbox70. Figure 5: Cross-classification test results with local pattern classifiers. We conducted whole-brain searches for candidate regions for shared neural processes between pain and rejection with 6-mm radius spherical searchlights around centre voxels. To determine the candidate regions, we conducted cross-classification tests (with leave-one-subject-out cross-validation) among the regions that accurately classify both pain (Heat-pain versus Warmth) and rejection (Ex-partner versus Friend). The cross-classification test consisted of the following steps: (i) A local classifier was trained and cross-validated separately for one condition, and (ii) the classifier was tested on the other condition in the same leave-one-subject-out cross-validation test sample. Here we thresholded all results at FDR q <0.05 ( P <0.0038) and visualized the 6-mm sphere coverage. PCC, posterior cingulate cortex; PHG, parahippocampal gyrus; RSC, retrosplenial cortex; TPJ, temporal parietal junction. The anatomical atlas was from the SPM anatomy toolbox [70] . Full size image As shown in Fig. 5 and Supplementary Table 2 , a number of regions showed significant cross-classification between pain and rejection (yellow in Fig. 5 ), implying shared representation at the local pattern level. These included the left parahippocampal and fusiform gyri, retrosplenial cortex, right TPJ, posterior cingulate cortex and striatum ( q <0.05, FDR corrected). Critically, none of these regions are primary ‘pain-processing’ regions [36] , [42] . Many other regions showed significant classification accuracy for both pain and rejection (orange in Fig. 5 ), but without significant cross-classification (that is, separate modifiability). Such regions did include those targeted by primary nociceptive afferents (for example, dACC, aINS and dpINS/S2). Distinct functional connectivity with dACC patterns In Study 2, we tested whether the distinct multivariate patterns for pain and rejection in the same local region of interest within the dACC are functionally connected to similar or different brain networks in a separate resting-state fMRI data set ( N =91; aim 3 ). In previous sections, we showed that the dACC was commonly activated by both pain and rejection ( Fig. 4a ), but we identified distinct multivariate fMRI patterns within the dACC, which were separately modifiable by pain and rejection ( Fig. 5 ). However, it is unknown whether these multivariate patterns for pain and rejection within the dACC connected to distinct brain circuits that correspond to distinct affective processes and large-scale brain networks. To examine this question, we used the Study 1 data to obtain dACC local-region patterns—defining the region as the portion of dACC that showed strong separate modifiability in the previous analyses—separately for Heat-Pain versus Warmth and Ex-partner versus Friend. This yielded dACC pain and dACC rejection multivariate patterns optimized to specifically detect each experience ( Fig. 6a ). Then, we calculated the expression of each pattern at each time point in the Study 2 resting-state fMRI data, yielding two ‘seed’ time courses based on the two patterns. In order to calculate the strength of expression of each pattern, we used the dot-product of a vectorized activation map within the dACC region of interest with the pattern classifier weights. Finally, we performed random-effects GLM analyses to estimate functional connectivity with each seed’s time course across the brain and the connectivity difference maps. 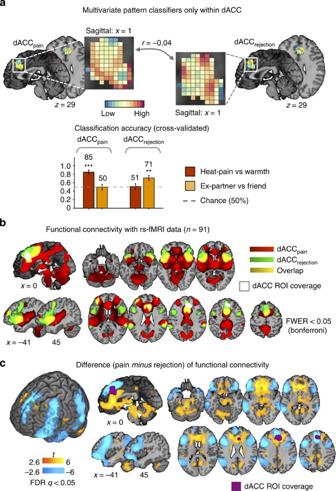Figure 6: Difference in functional connectivity patterns with dACC pattern classifiers for pain and rejection. (a) The multivariate pattern classifiers for pain and rejection within the dorsal anterior cingulate cortex (dACC) region-of-interest (ROI) (atop). The dACC ROI was defined by the searchlight analysis results presented inFig. 5, which showed that the dACC ROI contained information for both pain and rejection conditions, but the patterns were distinct and non-transferrable. Using the dACC ROI, we trained linear SVMs to discriminate pain and rejection from their respective control conditions, and tested on out-of-sample participants. The pattern weights were uncorrelated with each other,r=−0.04. The cross-validated (leave-one-subject-out) accuracy in two-choice classification tests demonstrated separate modifiability of the pattern classifiers (abottom). The dotted line indicates the chance level (=50%), and the error bars represent standard error of the mean across subjects. **P<0.01, ***P<0.001, binomial test. (b) Seed-based functional connectivity with dACC pattern classifiers for pain and rejection. Here seeds were pattern expression values (the dot-product of a vectorized activation map and SVM weights within dACC) for pain and rejection. The functional connectivity for each condition was calculated with independent resting-state fMRI data (n=91). These maps were thresholded at family-wise error rate (FWER)<0.05 using Bonferroni correction. Here we used Bonferroni correction instead of false discovery rate (FDR) because the latter provided too liberal thresholds for these functional connectivity patterns (uncorrectedP<0.03) and therefore yielded non-sensible maps. (c) Pairedt-test results between two seed-based functional connectivity patterns. The results were thresholded at FDR<0.05. Figure 6: Difference in functional connectivity patterns with dACC pattern classifiers for pain and rejection. ( a ) The multivariate pattern classifiers for pain and rejection within the dorsal anterior cingulate cortex (dACC) region-of-interest (ROI) ( a top). The dACC ROI was defined by the searchlight analysis results presented in Fig. 5 , which showed that the dACC ROI contained information for both pain and rejection conditions, but the patterns were distinct and non-transferrable. Using the dACC ROI, we trained linear SVMs to discriminate pain and rejection from their respective control conditions, and tested on out-of-sample participants. The pattern weights were uncorrelated with each other, r =−0.04. The cross-validated (leave-one-subject-out) accuracy in two-choice classification tests demonstrated separate modifiability of the pattern classifiers ( a bottom). The dotted line indicates the chance level (=50%), and the error bars represent standard error of the mean across subjects. ** P <0.01, *** P <0.001, binomial test. ( b ) Seed-based functional connectivity with dACC pattern classifiers for pain and rejection. Here seeds were pattern expression values (the dot-product of a vectorized activation map and SVM weights within dACC) for pain and rejection. The functional connectivity for each condition was calculated with independent resting-state fMRI data ( n =91). These maps were thresholded at family-wise error rate (FWER)<0.05 using Bonferroni correction. Here we used Bonferroni correction instead of false discovery rate (FDR) because the latter provided too liberal thresholds for these functional connectivity patterns (uncorrected P <0.03) and therefore yielded non-sensible maps. ( c ) Paired t -test results between two seed-based functional connectivity patterns. The results were thresholded at FDR<0.05. Full size image Figure 6a shows the multivariate pattern classifiers within dACC for pain and rejection and the cross-validated classification accuracy results, indicating that the dACC patterns for pain and rejection were distinct, r =−0.04, P =0.23 and separately modifiable by pain and rejection, as we expected. The whole-brain functional connectivity patterns for dACC pain and dACC rejection ( Fig. 6b ) and their difference map ( Fig. 6c ) showed that dACC pain and dACC rejection engage distinct functional connectivity patterns. For example, dACC pain showed stronger functional connectivity with thalamus, posterior insula, midbrain regions, ventral and anterior part of medial frontal regions, posterior cingulate cortex and cerebellum (yellow in Fig. 6c ), whereas dACC rejection was more strongly associated with ventral and dorsal lateral prefrontal cortex, parietal cortex, temporal pole and middle temporal lobe, dmPFC and TPJ (blue in Fig. 6c ). These networks correspond well to the regions with differential predictive weights for pain and rejection in Study 1, but they were identified using distinct methodology (resting-state fMRI connectivity) in an independent sample in the absence of overt pain or social rejection. The idea that there is substantial overlap in the neural representations of pain and rejection within core pain-processing regions such as dACC and aINS has been influential in various fields [1] , [47] . However, claims about shared representation in the previous studies have been based on findings of overlapping univariate fMRI activity between pain and rejection [2] , [4] , [5] , which is not anatomically specific enough to bear on the question of whether the underlying neural representations are similar. Here we used a more fine-grained analysis technique to demonstrate that the overlapping activity arises from distinct neural representations [18] . MVPA is more likely to reflect population codes across neurons [43] , [45] , [48] , as they have demonstrably greater sensitivity and specificity to particular types of mental events [17] , [31] , [32] . We demonstrate that multivariate patterns encoding the intensity of pain and rejection are separately modifiable [30] by showing that pain and rejection each influenced distinct, uncorrelated fMRI patterns at the whole-brain level and within ‘pain-processing’ regions. The criterion of separate modifiability, which is a stronger version of the classic ‘double dissociation’ logic, strongly implies the existence of distinct, non-shared neural representations for pain and rejection. The criterion also rules out a single-process interpretation (for example, based on salience, arousal or general aversiveness) of the fMRI multivariate patterns that we observed within and across regions. The logic of this claim is laid out more completely in ref. 30 , but it deserves a brief treatment here. We start by hypothesizing that the effects of both pain and rejection manipulations on dACC (or any other region discussed here) are related to a single process (for example, salience), and asking whether this hypothesis can be falsified with the separate modifiability criterion. Let us call the pain-related fMRI pattern in dACC ‘Pattern A.’ If rejection does not activate Pattern A, then there are three possibilities: (i) Pattern A does not reflect a common process engaged by both pain and rejection; (ii) Pattern A is not sensitive to the common process (for example, is too noisy) or (iii) rejection activates the common process too weakly. We can rule out (ii), because pain does activate Pattern A. Alternative (iii) is possible, although we note that subjective ratings of distress were comparable across pain and rejection ( Fig. 1b ). Now, let us consider that rejection activates Pattern B, but pain does not. If Pattern B also reflects activation of the same common process (for example, salience), then (iii) is ruled out, because rejection is demonstrated to be a more potent manipulation of Pattern B than pain. Thus, we conclude (i): ‘Pattern A does not reflect a common process engaged by both pain and rejection’. The same logic applies to Pattern B, and we can infer that neither pattern encodes a mental process that is shared by both pain and rejection. This is important in relation to recent literature interpreting fMRI activity in the dACC, aINS and other regions in terms of general processes (for example, both regions are part of the ‘salience network’ [24] ). Based on our findings and the separate modifiability logic, standard brain activation results may reflect non-specific, domain-general processes, but the multivariate patterns we identify here cannot. The existence of at least some neural dissociation of pain and rejection is trivial, in part because pain and rejection-related stimuli are initially processed in different sensory systems (that is, somatosensory versus visual), and also because they differ in their cognitive associations and implications. What is at stake, however, is whether core affective processes (for example, ‘pain affect’) are shared [2] , [47] , and whether the type of emotional distress elicited during pain is the same as that elicited during social rejection. Germaine to this issue, pain- and rejection-related multivariate patterns were uncorrelated and separately modifiable even within the regions thought to encode ‘pain affect,’ including the dACC and aINS. In addition, although both pain and rejection activate somatosensory areas, such as S2 and dpINS, we demonstrate here that they activate different multivariate patterns within these areas. Thus, together, the findings indicate separable neural representations that are co-localized at the gross anatomical level. It is important to consider how the multivariate patterns we identified might relate to those at more spatially precise levels of analysis, including optical imaging and single-unit recording. Ultimately, neural processes that underlie representations of mental constructs can be investigated at multiple levels of analysis. Among methods available in healthy humans, fMRI multivariate patterns may be particularly useful in inferring representational similarity [43] , as such patterns can be sensitive to population codes distributed across large numbers of individual neurons. FMRI multivariate patterns have obvious limitations in spatial resolution compared with single-unit recording [49] , in large part because blood-oxygen-level-dependent (BOLD) fMRI is sensitive to changes in microvascular beds that subserve many neurons, and the BOLD response thus acts as a spatial low-pass (blurring) filter sensitive to some, but not all, neuronal-level processes [48] , [50] . Because of the spatial blurring properties of fMRI, finding that two manipulations activate similar fMRI patterns does not necessarily imply similar neuron-level representations. However, finding dissociable fMRI patterns, as we did here, implies that the neuron-level population codes are different. An additional advantage of working at the fMRI pattern level is that fMRI can detect representations encoded across millions or billions of neurons, including interactions among large-scale brain networks, complementing approaches at finer spatial scales. It is also important to note that our findings do not imply that there are no shared representations anywhere in the brain. To the contrary, we identified a number of regions showing similar fMRI patterns for pain and rejection. However, these regions were located outside of core pain-processing brain systems [36] , [42] . Thus, shared representations may exist (proviso considerations outlined above), but they are not likely associated with nociceptive pain. Rather, they are likely to be broadly associated with processes related to context, memory, motivated action, social inferences, and/or endogenous regulation (for example, opioid response in striatum [13] , [51] ), among other processes. However, following the logic outlined above, we cannot claim that regions showing similar fMRI patterns are also similar at lower levels of analysis. The idea that pain and rejection share neurophysiological mechanisms has also been supported by neurochemical and pharmacological findings [11] , [13] , [52] , which at first may seem contradictory to our conclusion. However, similar neurochemical responses to pain and rejection (for example, endogenous opioids and oxytocin [12] ) may reflect common physiological regulatory responses to general aversive events (for example, stress). For example, the endogenous opioid system, implicated in both pain and rejection, also plays a key role in stress-induced analgesic effects [53] , which could explain the analgesic effects of acute experiences of social exclusion or separation [54] , [55] . In addition, the effects on rejection experience of ‘pain medications’ like acetaminophen [11] may be related to nonspecific neurochemical pathways for aversive affective states, such as the serotonin system [56] . Therefore, the involvement of common neuropeptides and regulatory mechanisms in both pain and rejection do not necessarily imply shared neural representations. More broadly, the multivariate pattern-based approach we use here has potential for identifying and targeting many types of affective processes more specifically, which could enable significant progress in understanding the structure of emotion and its regulatory mechanisms [9] and providing more specific and robust links between brain representations and psychopathology [57] . Importantly, our results do not imply that there is no functional relationship between pain and rejection, or that one cannot influence the other. In fact, such interactions may underlie, for example, the increased rate of pain disorders observed following emotional trauma [58] . Developing and using fMRI pattern-based markers that are sensitive and specific to different psychological experiences will provide new leverage points for examining their underlying neural processes, the regulatory effects on the processes, and inter-relationships among different psychological processes. This approach could ultimately contribute to developing tailored interventions for specific psychological problems by identifying unique components of each condition, and it could also guide diagnosis and treatment of mental disorders by providing provisional fMRI-based biomarkers for them [59] . This study also has implications for how networks are identified in fMRI studies. We showed that fMRI activity within localized anatomical regions (for example, the dACC region corresponding to Vogt’s anterior mid-cingulate zone [60] ) can be decomposed into two orthogonal multivariate patterns that, when used as ‘seed’ patterns in connectivity analyses, are associated with two distinct large-scale brain networks. This finding supports the idea that local regions such as dACC can contain multiple, distinct neural population codes [25] that encode distinct mental processes. Previous neuroimaging studies have generally assessed functional connectivity by averaging activity within localized ‘seed’ regions into a single variable, which implicitly assumes that all voxels within the ‘seed’ region share a common pattern of connectivity. Therefore, the current approach is qualitatively different from the traditional approach to functional connectivity, and has broad implications for network analysis in future fMRI studies. Previously, we published two papers using part of the current data set ( N =40, compared to N =60 currently) [4] , [32] . The first publication [4] reported overlapping fMRI activity across pain and rejection within many pain-processing regions, based on univariate GLM analyses. We interpreted these findings in terms of shared representations between pain and rejection. The co-localized representations may still point to important interactions between pain and rejection. However, the current findings at the multivariate pattern level suggest that the representations of pain and rejection are in fact distinct within and across regions. This conclusion, which differs from our previous interpretation of the data, does not result from the addition of 20 more participants (see Supplementary Fig. 7 ), but rather from the different level of analysis. The second previous publication [32] used part of this data set ( N =40) to test the cross-study sensitivity and specificity of an fMRI-based brain marker for experimental pain. The focus of the current study is qualitatively different: The previous paper [32] focused on the development of a new fMRI-based marker for pain, whereas the current study focuses on examining, and ultimately challenging, current notions of shared representation across social and physical pain. We believe the current study provides a more comprehensive picture of the relationship between pain and rejection than previous work, and provides a step towards a better understanding of the interaction between pain and rejection and developing tailored interventions for each of them. More specifically, the following analyses have been conducted only in the current study, not in the previous studies [4] , [32] : (i) we identified a multivariate fMRI pattern sensitive and specific to rejection; (ii) we demonstrated that the rejection pattern is qualitatively different from the pain pattern, and the rejection pattern did not respond to pain; (iii) we showed that pain and rejection yielded distinct multivariate patterns even in the overlapping regions activated by both pain and rejection; (iv) we identified brain regions with similar neural patterns for pain and rejection using a searchlight approach; and finally, (v) we showed that the distinct multivariate patterns for pain and rejection within the dACC engaged distinct functional brain networks using a separate resting-state data set ( N =91). The present study has limitations that should be addressed in future studies. Given that we used a five-point Likert scale for pain and emotion ratings and applied only two different intensity levels of stimulation for both pain and rejection, the multivariate patterns we identify here may not be sensitive to fine-grained differences in the subjective intensity of pain and rejection experience. Therefore, these multivariate patterns cannot be regarded as fully characterized representations of pain and rejection experience. We cannot also rule out the possibility that some of the activity in the multivariate patterns we identified could be related to response preparation, attention and other consequences, instead of mental representations central to the experience of pain and rejection. This is an important issue with all MVPA analyses and fMRI results in general [61] , and therefore future work will be required to identify fMRI representations of pain and rejection by characterizing their specificity and generalizability across different tasks, individuals and studies. Particularly, the stimuli used in the current social rejection task (for example, ex-partner photos) refer to past experience and only indirectly to present circumstance, whereas the somatic pain task elicits acute thermal pain. Therefore, other social rejection tasks eliciting acute feelings of exclusion (for example, the Cyberball game task [62] ) might provide a good additional comparison condition, although they are likely to elicit less intense rejection-related emotions than the current task. We also focused only on pattern-based classification across individuals because this approach is more stable and generalizable than the within-subject approach. However, identifying individual-specific multivariate patterns might also be informative about the relationship between pain and rejection. In conclusion, our results provide the first neuroimaging evidence that pain and rejection do not share neural representations within core pain-processing brain regions. Instead, the present findings suggest that pain and rejection are represented in distinct mesoscopic neural systems whose locations are conserved across individuals. This new approach, and the evidence for separately modifiable multivariate patterns for each type of ‘pain,’ can move the field beyond the search for shared processes across pain and rejection and provide a step towards identifying their unique components, developing tailored interventions for each of them, and obtaining a better understanding of the interactions between these two distinct affective processes. Participants Sixty healthy, right-handed participants (31 females, M age =20.8, SD age =3.0) completed the social rejection and somatic pain tasks while undergoing scanning with fMRI (Study 1). All participants experienced an unwanted romantic relationship break-up within the past 6 months, and indicated that they felt rejected when thinking about their break-up; all participants rated high on a 1 (not at all rejected) to 7 (very rejected) scale asking how rejected they felt when they thought about their rejection experience ( M =5.52, s.d.=1.08). Participants were recruited via flyers posted around Manhattan and advertisements posted on Facebook and Craigslist. The sample was comprised of 63% Caucasian, 15% Asians, 10% African Americans, 3% Hispanic and 8% other. All participants were native English speakers and received $175 for their participation. FMRI task data (for example, trial onset times) were lost for one participant. Thus, all imaging analyses were completed on 59 participants. The study was approved by the Columbia University’s Institutional Review Board. In addition, 91 healthy, right-handed participants (48 females, M age =20.8, SD age =2.8) completed the resting-state fMRI task (Study 2), separately from the social rejection and somatic pain tasks. The sample was comprised of 87% Caucasian, 4% Asians, 2% African Americans and 7% Hispanic. All participants were native English speakers and received $50 for their participation. The study was approved by the University of Colorado Boulder’s Institutional Review Board. All participants provided written informed consent. Participants were screened to ensure that they did not suffer from any neurological or psychiatric illness, experience chronic pain, take psychoactive medications, antihistamine or steroids, have metal in their bodies, or have a history of substance use or abuse. Social rejection task stimuli The social rejection task was designed after the following two lines of research: (i) fMRI research where photos provided by participants were used to elicit powerful emotions (for example, maternal love, romantic love and rejection) [51] and (ii) behavioural research where cues were used to recall autobiographical experiences of social rejection and to effectively reactivate distress related to social rejection [63] . The social rejection stimuli consisted of: (i) a headshot photograph of each participant’s ex-partner or a same-gendered friend with whom they shared a positive experience around the time of their break-up, and (ii) cue phrases displaying beneath each photograph that led participants to focus on a specific experience they shared with each person. Participants provided these cue phrases before the day of fMRI scanning using a procedure developed in prior research [64] : they first wrote a specific description of break-up experience with their ex-partner and positive experience with their friend. Subsequently, they created a cue-phrase to capture the gist of their experience. They were reminded of the cues they generated and the experiences they referred to on the day of scanning following established procedures. We cropped all images to ensure the total area of the photograph taken up by the face to be constant across Ex-partner and Friend images. Ratings of the picture quality and attractiveness by a group of ten individuals who were blind to the study goals and hypotheses indicated that the level of picture quality and attractiveness for each photograph did not differ between Ex-partner and Friend photographs. Somatic pain task stimuli For somatic pain stimuli, thermal stimulations were delivered to left volar forearm, consisting of two levels: non-painful (rated as level 2 on a 10-point scale by participants) versus very painful (rated as level 8 on a 10-point scale; near the limit of pain tolerance). With a calibration procedure [65] , we chose two temperatures on a participant-by-participant basis to be sure that the subjective pain intensity was constant across participants. We carried out the calibration task before the day of fMRI scanning. Pain calibration task Pain calibration consisted of 24 trials where participants rated the pain induced by thermal stimulation (10 °C s −1 ramp up, 7 s at target temperature, 10 °C s −1 ramp down) applied using a TSA-II Neurosensory Analyzer (Medoc Ltd) with a 16-mm thermode end-plate. Participants provided verbal ratings with a 0 (no sensation) to 10 (unbearable pain) scale. Thermal stimulations were applied in a fixed order through eight different, nonadjacent candidate skin sites on the participant’s left volar forearm. On each trial, we used an adaptive procedure to estimate temperatures corresponding to level 2, 5 and 8 (referred to as ‘low,’ ‘medium’ and ‘high’). For the estimation procedure, a linear regression model continuously fit the data collected up to that point during the calibration session with temperature as the independent variable and pain ratings as the dependent variable. Although the temperature–pain relationship is not perfectly linear, it is relatively robust to noise and can be fit with few observations. To make the calibration more robust to idiosyncratic behaviour on individual trials, we defined trials for which the absolute value of the residual based on the initial regression was greater than three times the median absolute deviation as outliers, and the model was re-fit without the outliers. The predicted low, medium and high temperature levels from the regression model were used to determine the temperature applied on the subsequent trial. Throughout the calibration, we used a fixed, counterbalanced order of heat-levels (high, medium or low). The order was chosen to equalize the transitional probabilities and to balance stimulation at high, medium and low temperatures across the eight skin locations. Pre-scan task training Before fMRI scanning, the experimenter described each step of the Social Rejection task (referred to as the ‘Photograph’ task to participants) and the Somatic Pain task (referred to as the ‘Heat’ task to participants). The experimenter explained that during the ‘Photograph’ task, participants would see photographs of their ex-partner and friend and cue-phrases beneath each photograph. Participants were asked to look directly at each photograph and reflect on the thoughts and emotions each photograph-cue pair elicited in them. During the Somatic Pain task, participants were asked to stare at the fixation cross during each trial and focus on the sensations elicited by the somatic stimulus. Participants were then instructed how to rate their affect following each type of trial and how to perform the visuospatial control task (see Fig. 1a for a detailed description of these tasks). Pain and affect ratings and post-scan questionnaire Following each trial, participants rated how they felt or the pain intensity they experienced using five-point Likert scales (1=‘very bad’ or ‘very painful’, 5=‘very good’ or ‘not painful’). For display purposes, these scores were reversed such that higher scores indicate worse mood or more pain ( Fig. 1b ). After participants exited the scanner, they were asked to write freely about the thoughts that came to mind regarding (i) their recent romantic relationship break-up and (ii) their positive experience with friends during the experiment in the fMRI scanner. Resting-state fMRI task During the resting-state fMRI task (5 min 34 s), participants were asked to relax with their eyes closed while remaining awake. FMRI acquisition and preprocessing for study 1 Whole-brain fMRI data were acquired on a GE 1.5 T scanner using a T2*-weighted spiral in-out sequence developed by Dr Gary Glover: repetition time (TR)=2,000 ms, echo time (TE)=40 ms, flip angle=84 and field of view=22 cm, 24 axial slices (3.5 × 3.5 × 4.5 mm 3 voxels) parallel to the anterior commissure-posterior commissure line. Structural data were acquired with a T1-weighted spoiled gradient-recalled sequence: 1 × 1 × 1 mm 3 , TR=19 ms, TE=5 ms, flip angle=20. Stimulus presentation and behavioural data acquisition were controlled using E-Prime software (PST Inc.). Structural T1-weighted images were co-registered to the mean functional image for each subject using the iterative mutual information-based algorithm implemented in SPM8 and manual adjustment of the starting point until the co-registration was satisfactory. Structural images were normalized to Montreal Neurological Institute space using SPM8. Before preprocessing of functional images, we removed the first four volumes to allow for image intensity stabilization. We also identified image-intensity outliers by computing the mean and standard deviation (across voxels) of intensity values for each image for all slices to remove intermittent gradient and severe motion-related artefacts present to some degree in all fMRI data. To identify outliers, Mahalanobis distances for the matrix of slice-wise mean and standard deviation values (concatenated) × functional volumes (time) were computed, and any values with a significant χ 2 value (corrected for multiple comparisons based on the more stringent of either FDR or Bonferroni methods) were considered outliers (less than 1% of images were outliers). Each time-point identified as outliers was included as a separate nuisance covariate in the first-level models. Then, functional images were corrected for differences in the acquisition timing of each slice and were motion (realignment) corrected using SPM8. The functional images were warped to SPM’s normative atlas using warping parameters estimated from co-registered, high-resolution structural images, interpolated to 2 × 2 × 2 mm 3 voxels, and smoothed with an 8-mm FWHM Gaussian kernel. This smoothing level has been shown to improve inter-subject functional alignment, while retaining sensitivity to mesoscopic activity patterns that are consistent across individuals [48] , [66] . FMRI acquisition and preprocessing for Study 2 Whole-brain fMRI data were acquired on a 3T Siemens Trio system (Siemens) with a 12-channel receiver head coil using a T2*-weighted functional EPI sequence: TR=2,000 ms, TE=29 ms, matrix size=64 × 64 × 33, flip angle=75, slice thickness=3.5 mm, field of view=24 cm. The first four volumes of the resting state data were first removed to allow for image intensity stabilization, followed by detection of frame-to-frame motion and intensity outliers using the Artifact Detection Toolbox. Skull stripping was then conducted using FSL’s Brain Extraction Tool (v5, FMRIB, Oxford, UK), followed by slice timing and motion correction (realignment). Functional images were smoothed with an 8-mm FWHM Gaussian kernel, and warped to the Montreal Neurological Institute template using FMRIB’s Linear Image Registration Tool. Using the Conn SPM toolbox [67] , data were temporally filtered using a band-pass filter to retain frequencies between 0.009 and 0.08 Hz. Non-neural sources of variance were removed by regressing out the six estimated head movement parameters ( x , y , z , roll, pitch and yaw) and their first temporal derivatives, the top five principal components from the signal averaged in the white matter and ventricles, and the frames identified as motion or intensity outliers, and the residual was retained for analyses of functional connectivity. Behavioural analysis Affect rating data ( Fig. 1b ) were analysed using a multi-level GLM analysis [68] ( http://wagerlab.colorado.edu/tools ). Linguistic Inquiry and Word Count software (LIWC [33] )—a word frequency-based text analysis tool—was used for text analysis ( Fig. 1c ). The written descriptions of participants’ stream of thoughts while watching their ex-partner’s photos were first filtered with the negative emotion category in the LIWC dictionary. Then, we calculated the word frequency for each negative emotion category using the sub-categories within the negative emotion category. First-level fMRI analysis for Study 1 SPM8 was used to conduct first-level GLM analyses by modelling task regressors corresponding to the 15-s photo/heat period, the 5-s affect/pain rating period and the 18-s visuospatial control task period. The fixation-cross epoch was designated the unmodelled baseline. For each task regressor, a Boxcar function was convolved with SPM8’s canonical haemodynamic response function. A high-pass filter of 180 s, which is well suited for pain and emotion elicited for longer duration, was then applied. Other regressors of non-interest (that is, nuisance variables) included (i) ‘dummy’ coding regressors for each run (intercept for each run); (ii) linear drift across time within each run; (iii) the six estimated head movement parameters ( x , y , z , roll, pitch and yaw; mean-centered) and their squares, their derivatives and squared derivative for each run (24 columns per run); (iv) indicator vectors for outlier time points identified based on their multivariate distance from the other images in the sample (see above); (v) indicator vectors for the first two images in each run. Voxel-wise statistical parametric maps for different trial types were calculated for each participant and then entered into MVPA ( Figs 2 , 3 , 4 , 5 ) or random-effects group GLM analyses ( Supplementary Fig. 3 ). Robust regression analysis was implemented for the group-level GLM analyses [69] . All results were thresholded at q <0.05, FDR corrected, two-tailed. Multivariate voxel pattern analysis We used linear SVMs [34] to train multivariate pattern classifiers for pain and rejection. For global pattern classifiers ( Figs 2 and 3 ), we first conducted feature selection to maximize predictability and generalizability of SVMs. A priori voxels associated with ‘pain’, ‘emotion’ and ‘social’ terms were selected based on the union of forward and reverse inference maps from the automated large-scale meta-analytic database of more than 5,800 published neuroimaging studies ( http://neurosynth.org [22] ; see Supplementary Fig. 1 ). The SVMs were implemented using custom Matlab code based on the Spider toolbox ( http://people.kyb.tuebingen.mpg.de/spider ). The pattern classifiers were trained on first-level contrast images for four different conditions (that is, Heat-Pain, Warmth, Ex-partner and Friend) to separately discriminate ‘Heat-Pain’ and ‘Ex-partner’ from the respective three other conditions using the one-against-all approach [34] (that is, Heat-pain against other conditions, including Ex-partner, and Ex-partner against other conditions, including Heat-pain). Bootstrap tests were conducted to provide P -values for voxel weights in order to threshold the classifier weights for display and interpretation ( Fig. 2b ). We constructed 10,000 bootstrap sample sets (with replacement) and ran SVMs on each. Two-tailed, uncorrected P -values were calculated for each voxel based on the proportion of weights above or below zero. With a leave-one-subject-out cross-validation procedure, we assessed classification accuracy of the SVM classifiers using the forced-choice test, where pattern expression values (that is, the dot-product of a vectorized activation image with the classifier weights) were compared for two conditions tested within the same out-of-sample individual, and the higher was chosen as pain or rejection. We calculated the accuracy for Heat-pain versus Ex-partner or Ex-partner versus Heat-pain, Heat-pain versus Warmth and Ex-partner versus Friend. We also conducted a multi-voxel pattern similarity analysis and a cross-classification test ( Figs 4 and 5 ), and functional connectivity analysis with resting-state fMRI data (Study 2). For more details of these analyses, see Results. How to cite this article: Woo, C.-W. et al. Separate neural representations for physical pain and social rejection. Nat. Commun. 5:5380 doi: 10.1038/ncomms6380 (2014).